Bottom-up synthesis of high surface area mesoporous crystalline silicon and evaluation of its hydrogen evolution performance As an important material for many practical and research applications, porous silicon has attracted interest for decades. Conventional preparations suffer from high mass loss because of their etching nature. A few alternative routes have been reported, including magnesiothermic reduction; however, pre-formed porous precursors are still necessary, leading to complicated syntheses. Here we demonstrate a bottom-up synthesis of mesoporous crystalline silicon materials with high surface area and tunable primary particle/pore size via a self-templating pore formation process. The chemical synthesis utilizes salt by-products as internal self-forming templates that can be easily removed without any etchants. The advantages of these materials, such as their nanosized crystalline primary particles and high surface areas, enable increased photocatalytic hydrogen evolution rate and extended working life. These also make the mesoporous silicon a potential candidate for other applications, such as optoelectronics, drug delivery systems and even lithium-ion batteries. Porous silicon (Si) has long been studied in many fields because of its special physical and chemical properties [1] . For example, porous Si has been deeply investigated in optoelectronics and sensors owing to its light-emitting properties, drug/gene delivery research has benefited from its high porosity and bio-compatibility [2] , [3] , [4] and in recent years, porous Si has also been evaluated as a Li-ion battery anode [5] , [6] . Porous Si is also considered a promising candidate for hydrogen-generating materials because of its chemical and photocatalytic/photoelectrochemical reactivities towards water [7] , [8] , [9] . After decades of development, there are two well-established methods to produce porous Si materials, namely, anodisation and stain etching [10] . However, both are top-down methods and suffer from low yield because of their corrosion nature, which generate pores by sacrificing Si. Therefore, high Si mass loss and the need for large quantities of toxic hydrofluoric acid (HF) make these methods high cost and inefficient. In recent years, a few alternative preparations have been reported. One type is magnesiothermic reduction of silica [11] , [12] . At elevated temperature, porous silica precursor is reduced by magnesium vapour, leaving the pore structure unchanged. Another approach utilizing sodiothermic reduction of zeolite NaY was reported to obtain higher surface area than the magnesiothermic method [13] . Both reduction processes, however, need pre-formed porous materials as the precursor, which makes the syntheses complicated. A few porous Si/C composite materials have been reported using a chemical vapour deposition method [5] , which is considered an effective bottom-up way to prepare nano-Si materials [5] , [14] . However, the Si unit in these materials is not porous, although the overall structure is porous and shows good electrochemical performance as a Li-ion battery anode [5] . More generally, the preparation of porous, especially mesoporous crystalline materials is a big challenge in material chemistry [15] , [16] . For common mesoporous crystalline metal oxide materials, numerous preparation methods have been reported utilizing many different synthesis techniques after the discovery of mesoporous materials in the 1990s (refs 16 , 17 , 18 , 19 , 20 ). In contrast, the syntheses of mesoporous elemental semiconductor materials are highly limited. This is probably due to the complications in the properties of precursors and differences in structure forming chemistry comparing with oxide-based mesoporous materials [15] . The first example of mesoporous germanium (Ge) materials, which were reported separately by Kanatzidis and colleagues using metathesis of GeCl 4 with K 4 Ge 9 , and Tolbert and colleagues through an alternative polymer form of (Ge 9 2− ) n were not been published until 2006 (refs 21 , 22 , 23 ). Both syntheses used surfactants as the pore formation templates. Utilizing reduction or metathesis of halogenides (for example, GeCl 4 ) is recognized as an effective solution synthesis of nanocrystalline group IV materials, such as the Ge materials discussed above [21] , [22] , [23] . This kind of metathesis reaction was later expanded to other porous germanium-rich chalcogenide frameworks [24] . A reduction reaction using lithium naphthanide as the reductant was also reported for making nanosized colloidal Ge particles [25] . In comparison, the first synthesis of Si nanocrystals, using SiCl 4 and RSiCl 3 (R=H and octyl) as the co-precursors, was reported by Heath [26] . Further development of this synthesis, using SiCl 4 as the only precursor, was initially reported by Kauzlarich and colleagues via Zintl salt metathesis [27] , [28] , [29] . Besides metathesis, other types of solution reactions were also used for Si nanocrystals via sodium naphthanide and hydride reagents [30] , [31] . However, unlike for Ge materials, solution synthesis of porous, crystalline Si materials has not yet been reported. Ideally, the preparation of porous materials should be facile and under ambient conditions. The tuning of surface area and pore size should be feasible and pores should be generated by easily removed templates. It is thus interesting that the only by-products of the reduction of halogenides are metal salts, which have been used as pore templates in some aerosol syntheses of porous oxide materials, and the influence of salt templates on particle formation was initially studied in depth by Zachariah and colleagues [32] , [33] . Such salts have excellent thermal stability, which helps maintain the pore structure during heat treatment, and excellent solubility in water, which makes their removal easy. These factors make the salts possible pore template candidates for porous Si materials. In this work, we report a bottom-up self-templating synthesis of mesoporous crystalline Si (mPSi) materials. The synthesis utilizes a Si halogenide precursor (SiCl 4 ), which may significantly decrease the cost of the process compared with using crystalline Si wafers as etching precursors. The pores are produced by salt by-products as self-forming templates rather than by chemical corrosion of Si, thus providing both high porosity and high mass yield. Moreover, the salt by-products can be easily removed by water instead of necessitating the use of harsh etchants such as HF, as is the case for other methods [11] . The primary particle size, pore size and specific surface area of mPSi can be tuned by adjusting the heat treatment temperature. The resulting mPSi materials show high surface areas, up to 580 m 2 g −1 , which to the best of our knowledge is the highest value of all reported mesoporous Si materials [10] , [11] , [13] , [34] . When used for hydrogen (H 2 ) generation by chemical reaction with KOH solution, this allows for an extremely high H 2 production rate of 0.095 g H 2 s −1 g −1 Si (1.33 mol H 2 s −1 mol −1 Si), which is 30 times higher than the previously reported result [7] . In addition, the high surface area, nanoscale primary particles and uniform mesopores of the mPSi materials allow for a significant improvement in photocatalytic H 2 evolution performance compared with the existing literature [9] . A high H 2 generation rate, up to 882 μmol H 2 h −1 g −1 Si, is obtained by the optimized mPSi material, and is accompanied by a long working life of at least 55 h. This result not only shows much improved performance over previous reports but also pushes the performance of Si to on par with the current best unloaded (co-catalyst-free) photocatalysts, demonstrating its viability for further investigation [35] , [36] , [37] . Synthesis and pore formation mechanism study Our synthesis route is based on SiCl 4 reduction utilizing salt by-products as pore templates. A schematic illustration of the proposed reaction pathway is shown in Fig. 1 . In contrast to other syntheses, which use reducing agents such as sodium naphthanide, we have found that employing the alkaline alloy NaK as a reducing agent leads to formation of amorphous rather than crystalline Si particles under ambient conditions [27] , [38] , [39] . Owing to their poor solubility in the solvent, salt by-products and Si are believed to precipitate out simultaneously, forming a solid matrix. The amorphous Si is converted to a crystalline framework composed of interconnected primary particles during the following heat treatment, with its growth being restricted by the salt. Similarly, the salt templates are also restricted by the Si network and thus have mostly uniform size. The material is then washed with water to remove the salt by-products, generating the final porous Si. The pore size, primary particle size, and surface area can be tuned by adjusting the heat treatment temperature. 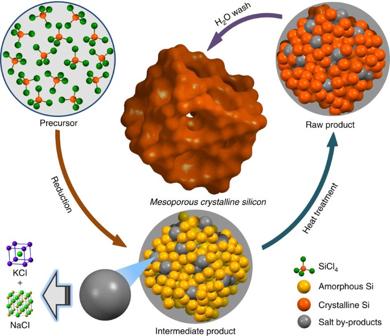Figure 1: Scheme of the synthesis route of mPSi. The pictures of the intermediate product and raw product are schematic illustrations that do not exactly reflect the real structures. Figure 1: Scheme of the synthesis route of mPSi. The pictures of the intermediate product and raw product are schematic illustrations that do not exactly reflect the real structures. Full size image To study the porous structure formation process, the raw product was isolated immediately after reduction and analysed. The raw product was composed of Si/salt matrixes that are considered the intermediate product, and some nanosized salt crystals separated from the Si/salt matrixes ( Supplementary Fig. 1 and Supplementary Discussion ). The peaks in the X-ray powder diffraction (XRD) pattern of the raw product ( Fig. 2a ) suggest the formation of crystalline KCl and NaCl, while the lack of observed Si peaks indicates the formation of amorphous Si. To examine the distribution of Si and salts in the matrixes, energy-dispersive X-ray spectroscopy (EDS) mapping was carried out on a cross-section of a single particle of the intermediate product ( Supplementary Fig. 2 ). K, Na, Cl and Si were found to be uniformly distributed throughout the cross-section of the particle, indicating the even dispersion of Si and salts in the matrix. The transmission electron microscopy (TEM) image of the intermediate product ( Fig. 2b ) shows that the mixture is composed of Si particles and salts. The corresponding selected-area electron diffraction pattern ( Fig. 2c ) also confirms the presence of crystalline salts. KCl crystallites (about 5–10 nm size) were observed between the amorphous Si particles in the high-resolution TEM (HRTEM) image ( Fig. 2d ). In addition, the Brunauer–Emmett–Teller (BET)-specific surface area of the intermediate product is 40 m 2 g −1 , which is much smaller than those of the final products ( vide infra ). The results discussed above confirm that the salt by-products form during the reduction and assist the pore formation, as schematically illustrated in Fig. 1 . 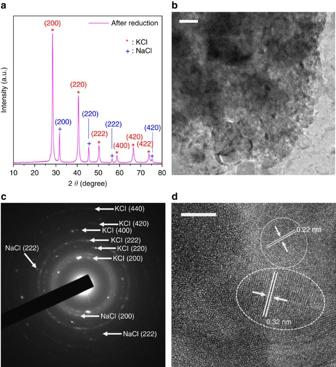Figure 2: Characterization of the intermediate products. (a) XRD pattern of the raw products obtained after reduction. The peaks of KCl (JCPDS Card number 41-1476) and NaCl (JCPDS Card number 05-0628) are labelled. Some of the NaCl peaks cannot be clearly distinguished owing to overlap with the KCl peaks. (b) Medium magnification TEM image of the intermediate products. Scale bar, 50 nm. (c) Selected-area electron diffraction (SAED) pattern of the intermediate products. The calculateddspacings from the SAED pattern are consistent with thed-spacing values for the corresponding planes of KCl and NaCl. (d) HRTEM image of the crystalline salt in the intermediate products. The lattice fringes of 0.32 and 0.22 nm labelled are consistent with thedspacings of the (2 0 0) and (2 2 0) planes of KCl, respectively. Scale bar, 5 nm. Figure 2: Characterization of the intermediate products. ( a ) XRD pattern of the raw products obtained after reduction. The peaks of KCl (JCPDS Card number 41-1476) and NaCl (JCPDS Card number 05-0628) are labelled. Some of the NaCl peaks cannot be clearly distinguished owing to overlap with the KCl peaks. ( b ) Medium magnification TEM image of the intermediate products. Scale bar, 50 nm. ( c ) Selected-area electron diffraction (SAED) pattern of the intermediate products. The calculated d spacings from the SAED pattern are consistent with the d -spacing values for the corresponding planes of KCl and NaCl. ( d ) HRTEM image of the crystalline salt in the intermediate products. The lattice fringes of 0.32 and 0.22 nm labelled are consistent with the d spacings of the (2 0 0) and (2 2 0) planes of KCl, respectively. Scale bar, 5 nm. Full size image Characterization of mPSi The mPSi materials were obtained by heat treatment of the raw product at different temperatures followed by removal of the salt templates by water. The resulting materials, namely, mPSi- X (where X is the heat treatment temperature in degrees Celsius), were then characterized. The mPSi-600 sample was studied first. The overall particle size of mPSi-600 ranges from 5 to 20 μm, as shown by SEM imaging ( Supplementary Fig. 3 ), and TEM images in Fig. 3a,b clearly show that the mPSi-600 has a disordered mesoporous structure. The Si framework consists of interconnected, multicrystalline primary particles with a size of below 10 nm. The crystallite size of mPSi-600 is around 3–5 nm, which is shown in the HRTEM image ( Fig. 3c ). This is consistent with the crystallite size (3.6 nm) calculated from the XRD pattern by the Debye–Scherrer equation ( Fig. 4a ). Nitrogen sorption analysis was also conducted for the mPSi-600 sample. The sorption isotherms shown in Fig. 4b are type-IV isotherm curves with an H1 hysteresis, indicating the presence of mesopores in the structure [40] . The narrow hysteresis loop with relatively steep and nearly parallel adsorption and desorption branches indicates that the mPSi-600 sample has good pore connectivity and a relatively narrow pore size distribution. The BET-specific surface area for mPSi-600 is 497 m 2 g −1 (1,152 m 2 cm −3 ). The pore size distribution (inset in Fig. 4b ) is centred around 10 nm, as calculated using the Barrett–Joynes–Halenda (BJH) method. This is consistent with the size of the salt templates seen in the HRTEM image of the intermediate product ( Fig. 2d ). The X-ray photoelectron spectrum (XPS) has peaks appearing around 99.8 and 103.5 eV, which are assigned primarily to Si (0) and Si (+4), respectively ( Fig. 4c ). The binding energies in between correspond to SiO x (0< x <2) [41] , [42] , [43] . Further detail on the XPS spectra is presented and discussed in Supplementary Fig. 4 , the Methods and the Supplementary Discussion . The surface oxygen content is determined to be around 32 atom% by XPS ( Supplementary Table 1 ), which is consistent with the oxygen content of 33 atom% by EDS spectroscopy ( Supplementary Fig. 3 ), suggesting that oxidation of mPSi-600 is uniform both on the surface and within the interior of the overall particle. The appearance of surface oxides, commonly observed in Si nanoparticles, is also verified by the Raman spectrum in which a peak shoulder appears between 300 and 450 cm −1 and is attributed to amorphous SiO x (0< x <2) and SiO 2 ( Fig. 4d ) [44] , [45] . The Raman spectrum of the mPSi-600 also shows a broad peak at 480 cm −1 , which indicates the presence of a layer of amorphous Si covering the crystalline core [46] . 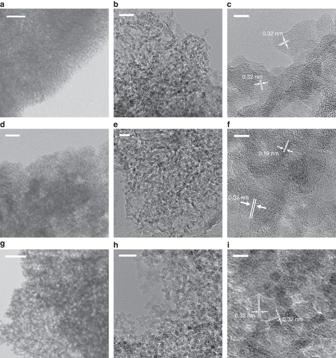Figure 3: Microscope images of mPSi materials. (a–c) Low, medium magnification TEM and HRTEM images of mPSi-600. The lattice fringes of 0.32 nm labelled are consistent with thed-spacing value of the (1 1 1) plane of silicon (JCPDS Card number 27-1402). Scale bar, 100, 20 and 5 nm, respectively. (d–f) Low, medium magnification TEM and HRTEM images of mPSi-700. The lattice fringes of 0.32 and 0.19 nm labelled are consistent with thed-spacing values of the (1 1 1) and (2 2 0) planes of silicon, respectively. Scale bar, 100, 20 and 5 nm, respectively. (g–i) Low, medium magnification TEM and HRTEM images of mPSi-820. The lattice fringes of 0.32 nm labelled are consistent with thed-spacing value of the (1 1 1) plane of silicon. Scale bar, 100, 20 and 5 nm, respectively. Figure 3: Microscope images of mPSi materials. ( a – c ) Low, medium magnification TEM and HRTEM images of mPSi-600. The lattice fringes of 0.32 nm labelled are consistent with the d -spacing value of the (1 1 1) plane of silicon (JCPDS Card number 27-1402). Scale bar, 100, 20 and 5 nm, respectively. ( d – f ) Low, medium magnification TEM and HRTEM images of mPSi-700. The lattice fringes of 0.32 and 0.19 nm labelled are consistent with the d -spacing values of the (1 1 1) and (2 2 0) planes of silicon, respectively. Scale bar, 100, 20 and 5 nm, respectively. ( g – i ) Low, medium magnification TEM and HRTEM images of mPSi-820. The lattice fringes of 0.32 nm labelled are consistent with the d -spacing value of the (1 1 1) plane of silicon. Scale bar, 100, 20 and 5 nm, respectively. 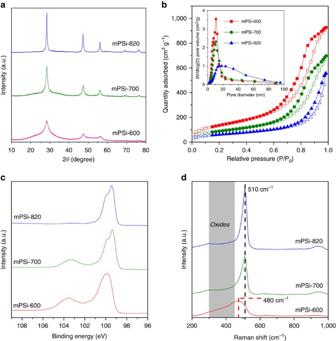Figure 4: Characterization of mPSi materials. (a) XRD patterns. (b) Nitrogen sorption isotherms and BJH pore size distributions (inset). (c) XPS spectra. (d) Raman spectra. Full size image Figure 4: Characterization of mPSi materials. ( a ) XRD patterns. ( b ) Nitrogen sorption isotherms and BJH pore size distributions (inset). ( c ) XPS spectra. ( d ) Raman spectra. Full size image By adjusting the heat treatment temperature to 700 and 820 °C, two different mPSi materials (mPSi-700 and mPSi-820) were also obtained and then characterized. As seen from SEM imaging ( Supplementary Fig. 3 ), the overall particle size of mPSi-700 is similar to that of mPSi-600, in the range of 5–20 μm, while the mPSi-820 shows both some larger particles of around 30 μm in size and some smaller particles. The TEM images of mPSi-700 and mPSi-820 ( Fig. 3d–i ) show similar disordered mesoporous structures to mPSi-600. However, the sizes of the primary particles are larger (~10 and 10–20 nm, respectively) than those of mPSi-600. The HRTEM images show that the crystallite sizes of mPSi-700 and mPSi-820 are 7–10 and 10–20 nm, respectively ( Fig. 3f,i ). This observation is also consistent with the crystallite size of 8.1 and 16 nm calculated from the XRD patterns. In the Raman spectra, the sharp Si peaks of mPSi-700 and mPSi-820 are at a higher Raman shift (510 cm −1 ) than the corresponding peak of mPSi-600, which suggests better crystallinity and lower amorphous Si content than in mPSi-600 ( Fig. 4d ) [46] , [47] , [48] . In addition, the lower signal intensity of the Si oxide bands between 300 and 450 cm −1 in the Raman spectra of mPSi-700 and mPSi-820 reveals that their oxide content is lower than that of mPSi-600. The oxygen concentrations of mPSi-700 (about 30 atom%) and mPSi-820 (about 8 atom%), determined from their EDS and XPS spectra ( Supplementary Fig. 3 and Supplementary Table 1 ), further indicate a lower oxide content. Since the Si oxides are composed of oxides from the native oxide layer and oxidation products by the water when removing the salts, the lower oxide contents of mPSi-700 and mPSi-820 could be due to their larger particles, better crystallinity and smaller surface area, which help limit oxidation when contacting air and water [49] . Figure 4b shows the nitrogen sorption isotherms of mPSi-700 and mPSi-820. BET-specific surface areas for mPSi-700 and mPSi-820 are 321 and 221 m 2 g −1 , respectively. The pore size distributions of mPSi-700 and mPSi-820 were calculated by the BJH method. The mPSi-700 shows a similar pore size distribution (centred at 10 nm) to that of mPSi-600, while the pore size for mPSi-820 is centred around 20 nm with a broad pore distribution ranging from 10 to 100 nm ( Fig. 4b , inset). Increased heat treatment temperature leads to Si grain growth and thus larger primary particle size, resulting in a smaller specific surface area. Photocatalytic hydrogen evolution of mPSi Anxiety about the increasingly serious global energy crisis and environment pollution makes producing H 2 , a clean fuel, more and more attractive [50] . Generating H 2 by using sunlight to split water via photocatalytic methods is particularly promising. Photocatalytic H 2 generation takes advantage of some of the unique abilities of semiconductors; after absorbing photons, electrons (holes) can be generated at the conduction band (valence band) of semiconductors. If the generated electrons and holes have enough energy to overcome the energetic barriers of both water reduction and oxidation and any overpotentials, photocatalytic water splitting will be realized [51] . Some oxide-based catalysts, such as TiO 2 , have been extensively studied since the 1970s and show good stability in this photocatalytic process. However, most of them show acceptable activity only under ultraviolet light owing to their large band gaps [51] , [52] . Although the band gaps of most sulphide-based catalysts (for example, CdS, ZnS-CuInS 2 and ZnS-AgInS 2 ) allow them to utilize visible light, the stabilities of these materials are poor [51] , [52] . This is mainly due to the reaction between sulphides and photogenerated holes in the catalysts. In addition, those with acceptable activity contain either the highly toxic element Cd or rare and expensive elements like In. Untill now, an efficient material for photocatalytic water splitting under visible light irradiation has not been discovered [53] . Si is one of the most promising candidates in the solar H 2 production area. The narrow 1.17 eV band gap of Si is appropriate for utilizing the solar spectrum, allowing it to capture photons up to the near-infrared region. In addition, it is the most abundant element on earth, precluding future problems of material scarcity. Moreover, thanks to the development of Si-based solar cells, the fundamental semiconductor physics and device fabrication processes of Si have been thoroughly studied. The development of nanostructured Si materials has also extended the use of Si into artificial photosynthesis, such as CO 2 fixation and H 2 generation [54] . Solar H 2 generation can take place via photoelectrochemical or powder photocatalytic systems. For photoelectrochemical solar H 2 evolution, photoelectrodes based on Si have been proved to be efficient [55] , [56] , [57] . However, the photoelectrochemical process usually needs external bias (provided by an external power supply) to surpass the overpotential, which hinders its application at large scales and introduces a parasitic energy cost. On the other hand, powder photocatalytic systems are considered better in large-scale solar water splitting owing to their simplicity [51] . Unfortunately, there are few reports on photocatalytic solar H 2 evolution by Si materials [9] . The limitation of such systems is mainly the small energy gap between the conduction band edge and the H + /H 2 potential, as well as the short working life commonly exhibited by conventional Si materials [9] , [58] . All mPSi materials showed wider band gaps (1.33–1.63 eV) than that of bulk Si (1.17 eV); band gaps were calculated according to ultraviolet–visible diffuse reflectance spectra ( Fig. 5a–c ). The expanded band gaps of the mPSi materials, which shift the conduction band to a more negative position and may thus facilitate H 2 evolution, are due to quantum confinement. The band gap crystallite size correlations are also consistent with previous theoretical calculations ( Supplementary Discussion ) [58] , [59] , [60] . The quantum-confinement effects were confirmed by photoluminescence spectroscopy ( Supplementary Fig. 5 and Supplementary Discussion ) [61] . 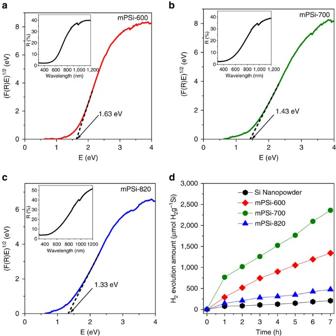Figure 5: Optical properties and photocatalytic performance. (a–c) Optical band gaps and ultraviolet–visible diffuse reflectance spectra (inset) of mPSi materials. (d) Typical reaction time course of the photocatalytic H2evolution of different unloaded porous Si materials and Si nanopowder under 300 W xenon light. Figure 5d shows the typical reaction time course of the photocatalytic H 2 evolution of different unloaded mPSi materials. All mPSi materials showed better photocatalytic H 2 evolution activity than commercially available Si nanopowder (191, 337 and 67 μmol H 2 h −1 g −1 Si in 7 h for mPSi-600, 700 and 820, respectively, versus 29 μmol H 2 h −1 g −1 Si in 7 h for commercial Si, Fig. 5e ). However, mPSi-600 showed a lower photocatalytic H 2 evolution rate (191 μmol H 2 h −1 g −1 Si in 7 h) than mPSi-700 (337 μmol H 2 h −1 g −1 Si in 7 h), although the surface area of mPSi-600 is much higher than that of mPSi-700. Figure 5: Optical properties and photocatalytic performance. ( a – c ) Optical band gaps and ultraviolet–visible diffuse reflectance spectra (inset) of mPSi materials. ( d ) Typical reaction time course of the photocatalytic H 2 evolution of different unloaded porous Si materials and Si nanopowder under 300 W xenon light. Full size image Refinement of mPSi-600 and photocatalytic performance Higher surface area can improve photocatalytic activity by providing more surface active sites. However, the photocatalytic activity also depends on the particle size, surface structure and crystallinity of the material, which greatly affect the rate of the charge generation, separation, migration and recombination steps [51] . Although mPSi-600 has a higher surface area, its photocatalytic H 2 evolution rate is lower than that of mPSi-700. The worse photocatalytic performance of mPSi-600 is probably because of its worse crystallinity and higher content of surface oxides, which may decrease the amount of effective surface active sites, prevent the migration of photogenerated charges and increase the recombination of the photogenerated electrons and holes [51] . To confirm this, mPSi-600 was further treated to remove the surface oxides, and the resulting refined material, namely, mPSi-600R, was then characterized. The overall particle size of mPSi-600R is similar to that of mPSi-600, as observed in the SEM image ( Supplementary Fig. 3 ). The TEM images ( Fig. 6a ) show a similar primary particle size to that of mPSi-600 (below 10 nm). More crystallites are observed in the HRTEM image ( Fig. 6b ) and the crystallite size ranges from around 2–5 nm, which is consistent with the result (3.2 nm) calculated from the XRD pattern ( Fig. 6c ). The sorption isotherm of mPSi-600R is similar to that of mPSi-600, having type-IV isotherm curves with an H1 hysteresis, and the BJH pore size distribution is also very similar ( Fig. 6d ). However, the BET surface area of mPSi-600R is slightly increased to 580 m 2 g −1 . The XPS spectrum ( Fig. 6e ) shows a strong decrease in the intensity of the peak at 103.5 eV as well some decrease in area corresponding to SiO x , which indicates a lower oxide content in the material. The oxygen concentration was found to be about 11 atom% based on EDS, which is consistent with the content found from the XPS spectrum ( Supplementary Fig. 3 and Supplementary Table 1 ). In the Raman spectrum ( Fig. 6f ), the sharpness of the major Si peak and its shift to 500 cm −1 , along with the much decreased intensity of the oxide peak at about 350 cm −1 , further confirm the less oxidized nature of mPSi-600R. The band gap of mPSi-600R was found to be 1.62 eV, as calculated according to its ultraviolet–visible diffuse reflectance spectrum ( Supplementary Fig. 6 ). A comparison of all band gaps calculated in this manner with values predicted based on theoretical models in the literature is presented in Supplementary Fig. 7 and the Supplementary Discussion . 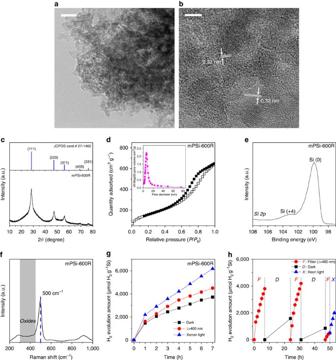Figure 6: Characterization and photocatalytic performance of mPSi-600R. (a,b) Medium magnification TEM and HRTEM images. The lattice fringes of 0.32 nm labelled are consistent with thed-spacing value of the (1 1 1) plane of silicon. Scale bar, 20 and 5 nm, respectively. (c) XRD patterns. (d) Nitrogen sorption isotherms and BJH pore size distribution (inset). (e) XPS spectrum. (f) Raman spectrum. (g) Comparison of H2evolution activities of mPSi-600R under different light conditions. (h) Cycling ability of mPSi-600R under different light conditions. Figure 6: Characterization and photocatalytic performance of mPSi-600R. ( a , b ) Medium magnification TEM and HRTEM images. The lattice fringes of 0.32 nm labelled are consistent with the d -spacing value of the (1 1 1) plane of silicon. Scale bar, 20 and 5 nm, respectively. ( c ) XRD patterns. ( d ) Nitrogen sorption isotherms and BJH pore size distribution (inset). ( e ) XPS spectrum. ( f ) Raman spectrum. ( g ) Comparison of H 2 evolution activities of mPSi-600R under different light conditions. ( h ) Cycling ability of mPSi-600R under different light conditions. Full size image The H 2 evolution performance of the refined sample was also tested. The photocatalytic activity of mPSi-600R was much better than that of the other mPSi samples, as summarized in Supplementary Fig. 8 and Supplementary Table 2 , allowing for an average H 2 generation rate of 882 μmol H 2 h −1 g −1 Si over 7 h of testing ( Fig. 6g ), which is comparable to the best reported unloaded photocatalysts (for example, MoS 2 /TiO 2 , (AgIn) x Zn 2 (1− x )S 2 , Cu 3 SnS 4 ) for solar H 2 evolution [35] , [36] , [37] . The photocatalytic activities of mPSi-600R under different illumination conditions were also studied. Unlike other tested samples, mPSi-600R showed an obvious reactivity towards water even under dark conditions ( Fig. 6g ). In general, the natural oxidation of Si by water, which generates H 2 , is slow [62] . The increased reaction rate of mPSi-600R is attributed to its enlarged surface area, which provides extra contact between the Si and water. This relationship between surface area and reaction rate is further demonstrated by a chemical reaction of mPSi-600R with KOH aqueous solution ( Supplementary Fig. 9 ). An extremely high average H 2 generation rate of 0.095 g H 2 s −1 g −1 Si (1.33 mol H 2 s −1 mol −1 Si) was obtained, which is about 30 times the highest reported result (0.003 g H 2 s −1 g −1 Si) [7] . In addition, mPSi-600R showed obvious photocatalytic reactivity under visible light ( Fig. 6g ). In contrast, no H 2 was generated under visible light by Si nanopowder [9] . The results of these tests, along with other H 2 generation tests mentioned previously, were found to be highly repeatable, as shown in Supplementary Figs 9 and 10 , and the Methods. The mPSi-600R also showed much longer working life compared with the previously reported result, in which the Si photocatalyst died after 5 h [9] . After 55 h of cyclic operation (three cycles, 21 h effective working time, Fig. 6h ), mPSi-600R still showed acceptable photocatalytic H 2 evolution rate (~400 μmol H 2 h −1 g −1 Si). To the best of our knowledge, the necessary cycle life for industrial application of photocatalytic H 2 evolution is not known. Nonetheless, our results show that porous Si photocatalysts have promising performance to go along with the other benefits of using Si, and are worth investigating further. The preparation of mPSi is composed of two key processes, which are reduction and heat treatment. The salt by-products are bi-functional during the synthesis. In the first step, these salts and Si are generated by the reduction of SiCl 4 and precipitate out owing to their poor solubility in toluene solvent. The exact nature of the precipitation process and following aggregation process is difficult to directly characterize; however, several factors are expected to direct these processes. According to the reaction equation, four equivalents of metal salt are generated for each equivalent of Si. In addition, NaK is a strong reducing agent, and SiCl 4 is a highly reactive precursor, so the reduction reaction is expected to be kinetically fast. Because of the larger quantity of salt formed and the fast kinetics of both salt and Si formation, the Si and salts simultaneously aggregate together to form a matrix. The salts then, in turn, act as pore templates; TEM images ( Fig. 2d ) clearly show that the salt crystals fill the space between Si particles, which later becomes the pores. Similar salt-templating processes have previously been reported in aerosol syntheses of porous oxide materials [32] , [33] . Although the salt is believed to serve as the pore template, the pores are not expected to perfectly replicate the shape of the salt crystallites. This is because the structure is formed by aggregation of similarly sized Si and salt particles, which produces extra voids between particles and can distort the final pore shape from the template shape. In the following heat treatment, the salts act as a pore filler to support the structure. They not only maintain the pores but also help restrict the growth of the Si framework owing to their good thermal stability. Concurrently, the growth of salt crystallites in mPSi-600 and mPSi-700 is significantly restricted by the Si framework, leading to similar pore sizes for these two samples. However, once the heating temperature reaches the melting points of the salts (melting point, KCl: 770 °C, NaCl: 801 °C), the salts melt and the growth of the Si becomes unrestricted. Thus, the resulting distribution of both Si primary particle size and pore size in mPSi-820 is not as uniform as in the other mPSi materials. This result indicates that the heat treatment temperature must be kept below 770 °C to obtain a uniform pore structure. After heat treatment, the salts can easily be removed by water, which makes the synthesis less complicated than other templating methods. The strong Si-Cl bonding (~380 kJ mol −1 ) makes the reduction reaction of SiCl 4 extremely harsh; only reductants that have enough reducing potential can cause this reaction to occur. According to the published results, only a few strong reducing reagents, such as sodium/sodium naphthanide and lithium/alkyllithium, work for this reaction. The NaK alloy used in this work is the only reagent so far that can create the desired porous crystalline Si materials. However, NaK is also an aggressive reagent and has similar limitations (for example, violent reaction with moisture) as the other reagents for SiCl 4 reduction. A milder/safer reagent that provides a balance between stability/safety and reactivity for the SiCl 4 reduction process would thus be a very desirable outcome from a future study. The mPSi materials possess several traits that make them attractive for photocatalytic H 2 generation. As an indirect band gap semiconductor, the absorption coefficient of Si is low in the visible light region. However, the mesoporous structure of the mPSi materials can help increase efficiency of light absorption and partially make up for this deficiency [63] , [64] . Critically, the demonstrated quantum confinement effects derived from the nanoscale crystallite sizes of mPSi lead to enlarged band gaps, which shift the conduction band to a more negative position and thus facilitate the H 2 evolution process [58] . In addition, the small particle sizes shorten the migration distances of photogenerated charges to the surface active sites, reducing recombination. The high carrier mobility of Si also benefits charge migration and facilitates photocatalysis [65] . Concurrently, the large surface area provides abundant reaction sites for H 2 evolution. These advantages grant the mPSi materials photocatalytic activities that are far superior to conventional Si nanoparticles. The surface state of the photocatalysts also plays a major role in their performance. The better H 2 evolution performance of mPSi-600R compared with mPSi-600 confirms that the surface state (here, oxide content) is very important to the photocatalytic activity, as the surface state can significantly change the amount of surface active sites and the migration of photogenerated charges [51] . On the basis of the convenient synthesis and promising H 2 evolution reactivity, the mPSi materials show great potential for full photocatalytic water splitting by pairing with an O 2 -evolution semiconductor (BiVO 4 , TiO 2 , even n -type Si) using a Z-scheme photocatalytic system [51] , [66] . In conclusion, we have developed a bottom-up synthesis of mPSi materials. The wet chemical synthesis avoids using external templates, so highly porous Si materials can be obtained entirely without etching. The oxide content can be significantly decreased by using a comparatively mild etching approach. This low-cost process is facile and efficient, and allows tuning of properties such as the surface area, pore size and primary particle size. Excellent chemical H 2 generation rate can be obtained, thanks to the high surface areas. More importantly, the high surface areas and mesoporous structure combined with the nanosized, crystalline primary particles enable much improved H 2 evolution rate and extended working life compared with the previously reported result. The performance is on par with the best reported unloaded photocatalysts for H 2 evolution [35] , [36] , [37] . Moreover, this synthesis method has a potential to be extended to other group IV elements to prepare corresponding porous materials. The advantages of this material also make it a possible candidate for other applications, such as optoelectronics, drug delivery systems and even Li-ion batteries. Preparation of mPSi The as-prepared NaK alloy (6 g) was added to 200 ml of toluene solution of anhydrous SiCl 4 (4 ml, Aldrich 99.998%) in a glovebox filled with Ar. (Caution: the NaK alloy is highly reactive and should be prepared with care under an Ar atmosphere.) The reaction mixture was stirred by magnetic stirring overnight under Ar. Twenty millilitres of diethyl ether solution of hydrogen chloride (2 M, Aldrich) was added to quench the remaining NaK. The raw products were collected by filtration and heated in a tube furnace at different temperatures (for example, 600, 700 and 820 °C, at 15 °C min −1 elevated rate) for 30 min under Ar flow. The yields of mPSi-600, 700 and 820 after calcination are nearly 100%, based on the stoichiometrically expected yield (1:4 Si:MCl ratio in the product, M=Na, K). The salt by-products were removed by washing with deionized (DI) water. The final product was obtained by filtration and dried under vacuum before use. The final yield of mPSi-600 is 91%. The yields of mPSi-700 and mPSi-820 are 89 and 88% based on Si. Refinement of mPSi-600 Typically, 400 mg of mPSi-600 was immersed in 50 ml 5wt% HF solution (with 1 ml ethanol added) for 1 h. The resulting material was collected by filtration and washed by degased DI water. The final product was dried at 60 °C under vacuum. Owing to its high sensitivity towards light and moisture, the mPSi-600R was stored in a light-shielded container under Ar. The yield of mPSi-600R is 71% based on mPSi-600. Characterization The samples were characterized on a Rigaku Dmax-2000 X-ray powder diffractometer (XRD) with Cu Kα radiation ( λ =1.5418 Å). The operating voltage and current were kept at 40 kV and 30 mA, respectively. The size and morphology of products were determined by a JEOL-1200 TEM, JEOL-2010 TEM and HRTEM, and FEI Nova NanoSEM 630 scanning electron microscope (SEM and EDS mapping). Owing to the sensitivity of the mPSi samples (specifically, mPSi-600 and mPSi-600R), the TEM samples were prepared by dropping the sample (dispersed in anhydrous hexane) onto the TEM grids inside the glovebox, and allowing the solvent to dry. The as-prepared grids were then transferred to the microscope facility in an air-tight container and were exposed to air for less than 1 min before TEM imaging. For the pore structure analysis, nitrogen sorption analyses were carried out at 77 K with a Micrometrics ASAP 2020 analyser (Micrometrics Instrument Corporation, Norcross, GA). Specific surface areas were calculated by the BET method using the adsorption branch in a relative pressure range from 0.04 to 0.25. The pore size distribution was calculated from the desorption branch of the N 2 isotherm with the BJH method. X-ray photoelectron spectroscopy (XPS) was conducted with a Kratos Analytical Axis Ultra XPS using monochromatic Al Kα radiation. High-resolution spectra were recorded with a pass energy of 20 eV in 0.1 eV steps. Binding energies were corrected with respect to the binding energy of the C 1 s peak at 284.8 eV. Raman spectroscopy was conducted with a WITec CMR200 confocal Raman instrument. Photoluminescence spectroscopy was performed using a Horiba Jobin Yvon Fluorolog 3–21 spectrometer. Diffuse reflectance ultraviolet–visible spectroscopy was performed by a Perkin-Elmer Lambda 950 spectrometer with a Labsphere DRA-CA-30I accessory. Fitting of XPS peak components Peak fitting was performed using the CasaXPS software, and was based on assumption of only Si and oxidized Si being present. The five Si oxidation states were fit with symmetric Gaussian/Lorentzian product peaks with a mixing parameter of 10 (mixing of 0/100 gives a pure Gaussian/pure Lorentzian line shape). Positions for the Si(0), Si(+1), Si(+2), Si(+3) and Si(+4) components were chosen based on literature values and allowed to vary by 0.1 eV during fitting, while the peak width was allowed to vary approximately within the bounds established by the literature [42] , [43] , [67] , [68] , [69] . Photocatalytic hydrogen evolution Photocatalytic H 2 evolution was performed in a gas-closed top window (quartz glass) Pyrex cell with a side septum neck for sampling, using a 300-W Xe lamp as the light source. The effective area of the cell is 40.7 cm 2 . gas samples (0.1 ml) were taken periodically and analysed for H 2 using a HP5890II gas chromatograph, with a thermal conductivity detector and a 15-m Rt-Mseive 5 A column (Restek). In all experiments, around 0.02 g of catalyst was added into the reaction cell and purged with argon for 30 min. Separately, 60 ml of DI water mixed with 10 ml of the sacrificial agent methanol (for scavenging the photogenerated holes) were also purged with Ar for 30 min. The water/methanol mixture was then added to the catalyst under Ar to begin the H 2 evolution reaction. Temperature for all photocatalytic reactions was kept at 25±5 °C. A controlled experiment was carried out before characterization, and no appreciable H 2 was detected without photocatalyst. To confirm the reproducibility of test results, the photocatalytic H 2 evolution tests of different samples and of mPSi-600R under different light conditions were repeated three times. All tests are largely consistent with one another, barring fairly minor variations ( Supplementary Fig. 10 ). The small differences observed come from minor weighing, sampling and instrumental errors. The average H 2 evolution comparison among all test samples is shown in Supplementary Fig. 8 . Supplementary Table 2 shows a summary of primary particle size, surface area, band gap and H 2 evolution rate of mPSi materials and Si nanopowder. Hydrogen generation by chemical reactions of mPSi-600R Measurements of H 2 generation over time were obtained by digital video analysis of gas evolution. Twenty-five millilitres of Schlenk flasks with a glass stopcock was used for the reactions. The H 2 generation rates demonstrated by chemical reaction of mPSi-600R with KOH aqueous solution are also largely repeatable (0.095, 0.070, 0.078 and 0.091 g H 2 s −1 g −1 Si, as measured in four separate tests, Supplementary Fig. 9 ). The reactions went to completion within 4 s, allowing the total H 2 generation amount to be compared with the stoichiometric amount. Total H 2 yields in terms of mol H 2 mol −1 Si are in the range of 1.6–1.8 mol H 2 mol −1 Si. This is smaller than the stoichiometric yield (2 mol H 2 mol −1 Si) owing to mPSi-600R containing some Si oxides, which has been proved by other characterization. As oxidized silicon can produce less or no hydrogen by reaction with KOH aqueous solution (depending on its degree of oxidation), it is reasonable that mPSi-600R has a below-stoichiometric H 2 yield. The average reaction rate of the full reaction process is 0.04–0.07 g H 2 s −1 g −1 Si (0.56–0.98 mol H 2 s −1 mol −1 Si). How to cite this article: Dai, F. et al. Bottom-up synthesis of high surface area mesoporous crystalline silicon and evaluation of its hydrogen evolution performance. Nat. Commun. 5:3605 doi: 10.1038/ncomms4605 (2014).